Calcium modulates force sensing by the von Willebrand factor A2 domain von Willebrand factor (VWF) multimers mediate primary adhesion and aggregation of platelets. VWF potency critically depends on multimer size, which is regulated by a feedback mechanism involving shear-induced unfolding of the VWF-A2 domain and cleavage by the metalloprotease ADAMTS-13. Here we report crystallographic and single-molecule optical tweezers data on VWF-A2 providing mechanistic insight into calcium-mediated stabilization of the native conformation that protects A2 from cleavage by ADAMTS-13. Unfolding of A2 requires higher forces when calcium is present and primarily proceeds through a mechanically stable intermediate with non-native calcium coordination. Calcium further accelerates refolding markedly, in particular, under applied load. We propose that calcium improves force sensing by allowing reversible force switching under physiologically relevant hydrodynamic conditions. Our data show for the first time the relevance of metal coordination for mechanical properties of a protein involved in mechanosensing. In response to vascular lesions, platelets are stimulated to secure bleeding arrest by formation of a platelet plug. In the high-shear environment found in the microvasculature or stenosed arteries, the adhesion of platelets critically depends on interactions with the plasma glycoprotein von Willebrand factor (VWF). This factor recruits platelets to sites of vascular damage by interacting with collagen and the platelet receptor GPIbα [1] , [2] . VWF is synthesized and assembled into large, disulphide-bonded multimers in endothelial cells and platelet precursor megakaryocytes, and the multimer size of VWF determines its platelet-adhesive potency in a force-dependent manner. VWF circulates in the bloodstream as a series of multimers with a broad size distribution, whereas ultra-large VWF multimers (ULVWFs) are stockpiled in specialized storage organelles of endothelial cells and platelets [3] from which they are released in response to thrombogenic stimuli. The circulating pool of smaller VWF multimers depends on high shear forces to become activated for platelet recruitment, whereas ULVWF molecules, which may exceed 50,000 kDa in size [4] , avidly bind to their platelet receptor GPIbα even at low shear stress. Upon secretion, ULVWF multimers remain initially attached to the cell surface, where they are then progressively cleaved at the Tyr1605–Met1606 scissile bond located within its A2 domains into smaller, less adhesive multimers by a specialized VWF cleaving protease ADAMTS-13 (a disintegrin and metalloproteinase with thrombospondin type 1 motif, member 13) [5] , [6] . This proteolytic regulation represents a critical 'inactivation' process that precludes the formation of spontaneous platelet-rich thrombi that may occlude the microvasculature. Accordingly, defective regulation of VWF multimer size is the cause of severe disorders. Depletion of high-molecular-weight multimers because of mutations in the A2 domain that presumably increase susceptibility to proteolysis by ADAMTS-13 cause a bleeding tendency, named type 2A von Willebrand disease [7] , [8] , [9] . In contrast, accumulation of ULVWFs in circulation because of a congenital or acquired deficiency of ADAMTS-13 is the cause of thrombotic thrombocytopenic purpura, which is characterized by severe thrombosis in the microvasculature [8] , [9] , [10] . Regulation of VWF multimer size is unique in its dependence on hydrodynamic shear forces. Recent studies show that the Tyr1605–Met1606 scissile bond is buried inside the VWF-A2 domain, which must be unfolded to become a substrate for ADAMTS-13 (refs 11 , 12 , 13 ). Consistent with binding of an unfolded conformation of A2, a crystal structure of the non-catalytic DTCS domains of ADAMTS-13 described an elongated, discontinuous linear array of three VWF-binding exosites [14] . Very recently, Zhou et al . [15] identified a calcium-binding site in the crystal structure of a disulphide-engineered A2 domain and demonstrated that calcium binding impedes proteolytic processing by ADAMTS-13 in static cleavage assays. Here we report the crystal structure of the wild-type (wt)-A2 domain with bound calcium, and show that calcium binding markedly increases its thermodynamic and mechanical stability and provides the capability to refold despite tensile forces. The crystal structure of the A2–Ca 2+ complex together with molecular dynamics simulations reveals a long-range stabilizing effect of calcium on the scissile strand. This finding raises the question whether calcium modulates the force-sensing function of A2 and hence regulates sensitivity to ADAMTS-13. Using optical tweezers we probed, at the single-molecule level, how calcium affects the mechanical response of A2 under tensile forces. We find that calcium has a dual role in mechanosensing: by increasing force resistance of A2 and stabilizing an intermediate fold that promotes refolding under applied load. Our data indicate a direct role of metal ions in modulating the functions of a protein force sensor. 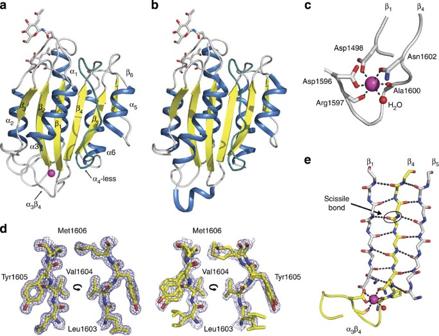Figure 1: The calcium-binding site of A2 affects scissile strand dynamics. Crystal structures of calcium-bound wt-A2 (a) and, for comparison, calcium-free A2 (b; protein data bank (PDB) accession code3GXB, ref.12) are shown in cartoon representation. The central β-sheet (yellow) is encircled by α-helices (blue). Magenta, calcium ion; dark cyan, α4-less loop; sticks,N-acetyl-D-glucosamine (GlcNAG) on residues Asn1515 and Asn1574. Both structures are similar, except for the clear rearrangement of the α3β4-loop (a 310helix in calcium-free A2) that forms most of the calcium-binding site. (c) Close-up of the calcium-binding site of A2. The calcium ion is coordinated by the α3β4-loop, Asp1498 and a water molecule (red sphere). Key side chains are shown in stick representation. (d) Close-ups of the scissile bond region in calcium-bound A2 (left) and calcium-free A2 (PDB accession code3GXB, ref.12; right) show, respectively, a single, well-defined conformation and local disorder with multiple side and main-chain conformations. Electron density is contoured at 0.6eÅ−3. (e) Backbone representation of the β4-scissile strand (yellow) and neighbouring strands illustrating how calcium interlocks β4with β1via coordination by Asp1498 and Asn1602. Crystal structure of calcium-bound VWF-A2 We obtained well-diffracting crystals of the wt VWF-A2 domain in complex with calcium ion and determined its structure at 1.7 Å resolution ( Table 1 ). The crystal asymmetric unit contains three A2 molecules that are essentially identical and comprise residues 1,478–1,674; we do not observe interpretable density for amino-terminal residues 1,478–1,493, most likely because of flexibility. The overall arrangement of A2, like observed previously [12] , [15] , largely follows the canonical α/β topology of VWA domains with a parallel central β-sheet (β 1 –β 6 ), flanked on one side by an antiparallel edge strand (β 3 ) and encircled by amphipathic α-helices (α 1 –α 6 ) that pack against the two faces of the hydrophobic sheet ( Fig. 1a,b ). A2 is set apart from all other structurally characterized members of the VWA fold by its lack of the α 4 -helix, which is substituted by an elongated loop referred to as the α 4 -less loop [12] . The α 4 -less loop appears flexible: it adopts distinctly different conformations in the three independent A2 molecules in our structure and in the structure of calcium-free A2. Unlike the structurally homologous neighbouring domains A1 and A3, and in accordance with its role in the reduction of VWF multimer size, A2 is devoid of an intramolecular disulphide bond between N- and C-terminal cysteine residues. Instead, C-terminal residues Cys1669 and Cys1670 form a buried vicinal disulphide bond at the C-terminus of helix α 6 . The cleavage site for ADAMTS-13 between residues Tyr1605 and Met1606 is centrally positioned in β 4 , deeply buried in the middle of the hydrophobic core and inaccessible in the native conformation. The calcium ion predominantly interacts with the α 3 β 4 -loop that, intriguingly, immediately precedes the β4-strand bearing the scissile bond. Table 1 Data collection and refinement statistics. Full size table Figure 1: The calcium-binding site of A2 affects scissile strand dynamics. Crystal structures of calcium-bound wt-A2 ( a ) and, for comparison, calcium-free A2 ( b ; protein data bank (PDB) accession code 3GXB , ref. 12 ) are shown in cartoon representation. The central β-sheet (yellow) is encircled by α-helices (blue). Magenta, calcium ion; dark cyan, α 4 -less loop; sticks, N -acetyl- D -glucosamine (GlcNAG) on residues Asn1515 and Asn1574. Both structures are similar, except for the clear rearrangement of the α 3 β 4 -loop (a 3 10 helix in calcium-free A2) that forms most of the calcium-binding site. ( c ) Close-up of the calcium-binding site of A2. The calcium ion is coordinated by the α 3 β 4 -loop, Asp1498 and a water molecule (red sphere). Key side chains are shown in stick representation. ( d ) Close-ups of the scissile bond region in calcium-bound A2 (left) and calcium-free A2 (PDB accession code 3GXB , ref. 12 ; right) show, respectively, a single, well-defined conformation and local disorder with multiple side and main-chain conformations. Electron density is contoured at 0.6 e Å −3 . ( e ) Backbone representation of the β 4 -scissile strand (yellow) and neighbouring strands illustrating how calcium interlocks β 4 with β 1 via coordination by Asp1498 and Asn1602. Full size image Calcium binding affects scissile bond dynamics The calcium ion is coordinated by four residues from the α 3 β 4 -loop and a single residue, Asp1498, located in strand β 1 near the N-terminus of the domain ( Fig. 1c ). The coordination motif of the class II calcium-binding site involves main-chain carbonyl oxygen atoms of Arg1597 and Ala1600 and the side chain of Asn1602, as well as the monodentate carboxylate ligands of side chains of Asp1498 and Asp1596. A single water molecule completes the octahedral coordination sphere. The coordination stereochemistry is in very good agreement with reference values ( Supplementary Table S1 ) [16] , [17] , [18] and together with the refined crystallographic parameters confirms calcium as the metal ion. As commonly observed for VWF-A domains [19] , [20] , α 3 β 4 is additionally anchored by the side chain of the highly conserved Arg1597, which engages in ionic interactions with the carboxylate side chain, and hydrogen bonds to the main-chain carbonyl, of Asp1498 ( Supplementary Fig. S1a–c ). Binding sites for divalent metal ions have been described for other proteins containing VWA domains. In I-domains of the integrin family of cell adhesion receptors, metal coordination by a metal ion-dependent adhesion site, located at the 'top' of the domain, has an important role in ligand binding [21] , [22] , [23] . In contrast, the calcium-binding site of the A2 domain, which is strictly conserved in mammals ( Supplementary Fig. S1d ), is located at the 'bottom' of a VWA domain and, in the absence of known VWF-A2 ligands, appears to have a functional role different from ligand binding. Although leaving the overall structure unchanged, calcium binding leads to a substantial rearrangement of the α 3 β 4 -loop ( Supplementary Fig. S1e ). The calcium ion is located as far as 16 Å away from the peptide bond cleaved by ADAMTS-13, but, nevertheless, clear differences exist between the calcium-bound and calcium-free structures with respect to the dynamics of residues near the scissile bond. In the calcium-free structure, alternate backbone geometries and multiple side chain conformations exist for several residues within scissile strand β 4 (ref. 12 ). In contrast, for calcium-bound A2 we observe a well-defined main-chain trace and, with exception of Leu1603, single side chain conformations throughout the scissile strand ( Fig. 1d ). These apparent local differences in conformational flexibility cannot be attributed to differences in core packing ( Supplementary Fig. S2 ). Molecular dynamics simulations show that the absence of calcium induces flexibility in the calcium-binding α 3 β 4 -loop and that this mobility propagates to the two central strands β 1 and β 4 including the scissile bond ( Supplementary Fig. S3 ). It appears therefore that extension of the hydrogen bond network between β 1 and β 4 with a pair of strong ionic and ion–dipole interactions, provided by the calcium-coordinating residues Asp1498 and Asn1602 ( Fig. 1e ), rigidifies the scissile bond region. Electrostatic repulsion modulates native A2 domain stability We used a thermal denaturation assay to assess the effect of calcium on the stability of the VWF-A2 domain by monitoring protein unfolding with an environment-sensitive fluorescent dye [24] , [25] in the presence and absence of calcium. A marked increase in thermal stability was observed after addition of calcium ions, which shifted the T m of A2 in a concentration-dependent manner from 45 to 64 °C ( Fig. 2a ). Analysis of the concentration-dependent T m shift [26] observed upon titration with calcium ( Fig. 2b ) suggests that VWF-A2 binds calcium with an apparent K D of 0.2±0.04 (s.e.m.) μM. Comparison with unfolding curves obtained for a series of different divalent cations demonstrates that the observed stabilizing effect is specific for calcium ( Fig. 3 ). Importantly, a consistent shift in T m upon addition of calcium is also observed for constructs of A2 that contain its flanking domains A1 and/or A3, whereas no significant shift in T m is observed for the isolated A1 or A3 domain ( Fig. 2c ). These data show that VWF-A2, both in isolation and in the relevant domain context of full-length VWF, is stabilized by a metal ion binding-site that displays high affinity and specificity for calcium. 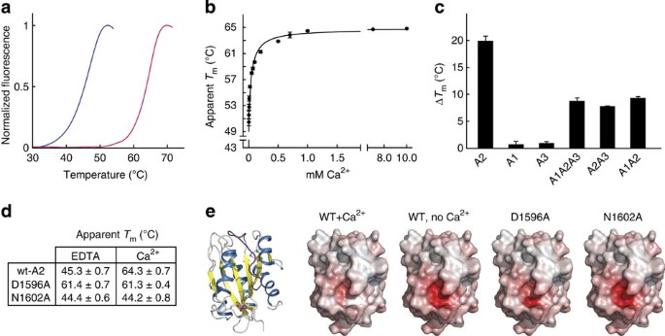Figure 2: Calcium stabilizes the native conformation of A2. (a) Thermofluor stability assays were performed with monomeric A2 in buffer without (blue) or with (red) 1 mM CaCl2. Curves were normalized to maximum fluorescence signal. Data show representative curves of triplicate experiments. (b) Calcium binds A2 with high affinity and stabilizes A2 in a concentration-dependent manner. Apparent melting temperatures were extracted from the mid-point of the unfolding transitions. Error bars represent s.d. (c) Comparison of the difference in apparent melting temperature for individual VWF-A domains with native tandem constructs determined in the presence and absence of 1 mM CaCl2. A consistent shift of the unfolding temperature is only observed if A2 is part of the construct. Bar graphs represent meanTmdifferences with respect to conditions containing EDTA (n=3). Error bars represent s.d. (d) Summary of unfolding temperatures (±s.d.) in the presence and absence of calcium. (e) Comparison of surface electrostatic potentials of wt-A2 and the D1596A and N1602A mutants. As reference, a ribbon model is shown in the same orientation. Electrostatic potentials were calculated on the solvent-accessible surface and contoured at −15 (red) to +15 (blue)kTe−1(wherekis the Boltzmann constant,Tis temperature andeis elementary charge). The strongly negatively charged surface pocket forms the calcium-binding site. Thermal stability correlates with neutralization of electrostatic repulsion in the calcium-binding pocket. Figure 2: Calcium stabilizes the native conformation of A2. ( a ) Thermofluor stability assays were performed with monomeric A2 in buffer without (blue) or with (red) 1 mM CaCl 2 . Curves were normalized to maximum fluorescence signal. Data show representative curves of triplicate experiments. ( b ) Calcium binds A2 with high affinity and stabilizes A2 in a concentration-dependent manner. Apparent melting temperatures were extracted from the mid-point of the unfolding transitions. Error bars represent s.d. ( c ) Comparison of the difference in apparent melting temperature for individual VWF-A domains with native tandem constructs determined in the presence and absence of 1 mM CaCl 2 . A consistent shift of the unfolding temperature is only observed if A2 is part of the construct. Bar graphs represent mean T m differences with respect to conditions containing EDTA ( n =3). Error bars represent s.d. ( d ) Summary of unfolding temperatures (±s.d.) in the presence and absence of calcium. ( e ) Comparison of surface electrostatic potentials of wt-A2 and the D1596A and N1602A mutants. As reference, a ribbon model is shown in the same orientation. Electrostatic potentials were calculated on the solvent-accessible surface and contoured at −15 (red) to +15 (blue) kTe −1 (where k is the Boltzmann constant, T is temperature and e is elementary charge). The strongly negatively charged surface pocket forms the calcium-binding site. Thermal stability correlates with neutralization of electrostatic repulsion in the calcium-binding pocket. 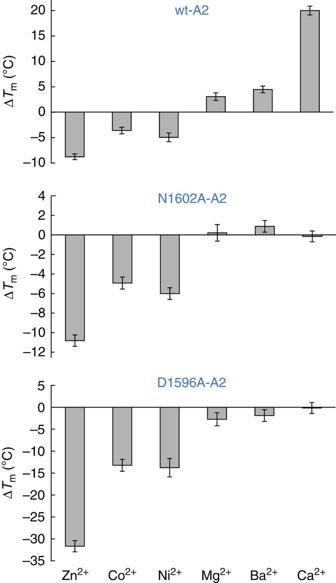Figure 3: Thermal stabilization of A2 is specific for calcium. Thermofluor stability assays were performed with the monomeric wt-A2 or the calcium-binding-deficient mutants N1602A and D1596A in buffer with 1 mM CaCl2, 20 mM BaCl2, 10 mM MgCl2, 10 mM CoCl2, 10 mM NiCl2or 10 mM ZnCl2. Bar graphs represent meanTmdifferences with respect to conditions containing EDTA (n=3). The qualitative similarity of the data obtained for wt-A2 and both mutants with respect to the effect of Co2+, Ni2+and Zn2+indicates that the destabilizing effect observed for these metal ions does not result from competition with the calcium site. Error bars represent s.d. Full size image Figure 3: Thermal stabilization of A2 is specific for calcium. Thermofluor stability assays were performed with the monomeric wt-A2 or the calcium-binding-deficient mutants N1602A and D1596A in buffer with 1 mM CaCl 2 , 20 mM BaCl 2 , 10 mM MgCl 2 , 10 mM CoCl 2 , 10 mM NiCl 2 or 10 mM ZnCl 2 . Bar graphs represent mean T m differences with respect to conditions containing EDTA ( n =3). The qualitative similarity of the data obtained for wt-A2 and both mutants with respect to the effect of Co 2+ , Ni 2+ and Zn 2+ indicates that the destabilizing effect observed for these metal ions does not result from competition with the calcium site. Error bars represent s.d. Full size image Thermal stability assays with alanine mutants of calcium-coordinating residues Asp1596 and Asn1602 (the D1498A mutant could not be expressed, likely because its above-mentioned interaction with Arg1597 is essential for domain stability) gave intriguing results. Despite its inability to bind calcium, the D1596A mutant shows thermal stability comparable with wt-A2 in the presence of saturating calcium concentrations. In contrast, N1602A unfolds at a temperature similar to wt-A2 in the absence of calcium ( Fig. 2d ). Apparently, loss of thermal stability because of the absence of a positively charged calcium ion can be compensated by the removal of the negatively charged side chain of Asp1596. These results suggest that neutralization of electrostatic repulsion by binding of calcium to the highly negatively charged calcium-binding pocket ( Fig. 2e ) is a prominent factor of domain stability. ADAMTS-13 sensitivity parallels thermal stability Cleavage of A2 by ADAMTS-13 requires partial unfolding of A2 to uncover the buried cleavage site [13] . The cleavage rate of any proteolysis reaction will involve a balance between the accessibility of the cleavage site, that is, substrate availability, and the efficiency of the cleavage reaction. To discern these effects, we performed cleavage experiments with both a folded A2 domain and a calcium-binding deficient, unstructured substrate polypeptide comprising C-terminal residues Asp1596–Arg1668 of A2 (ref. 15 ) fused to human growth hormone (hGH–VWF73). As ADAMTS-13 requires divalent metal ions for activity, we performed experiments either in the presence of 5 mM calcium or 5 mM barium, which similarly activates ADAMTS-13 (refs 5 , 6 ), but only marginally stabilizes A2 ( Fig. 3 ). Proteolysis of the folded wt-A2 domain or the calcium-binding-deficient mutants D1596A and N1602A reveals a clear correlation between thermal stability and ADAMTS-13 sensitivity ( Fig. 4a ). In the presence of calcium low cleavage levels of wt-A2 were observed, whereas cleavage occurred readily when calcium was substituted by barium ( Fig. 4b ). Consistent with the thermal stability data, cleavage levels for the thermostable D1596A mutant were similar to calcium-stabilized wt-A2, no matter whether cleavage conditions contained calcium or barium, thus confirming that stability of this mutant is independent of metal coordination. The thermolabile mutant N1602A was cleaved efficiently and at a similar rate as wt-A2 in the absence of calcium ( Fig. 4a,b ). These data demonstrate that calcium binding by native A2 decelerates cleavage under static conditions and supports a functional role of calcium in stabilizing the scissile bond in its native, concealed conformation. 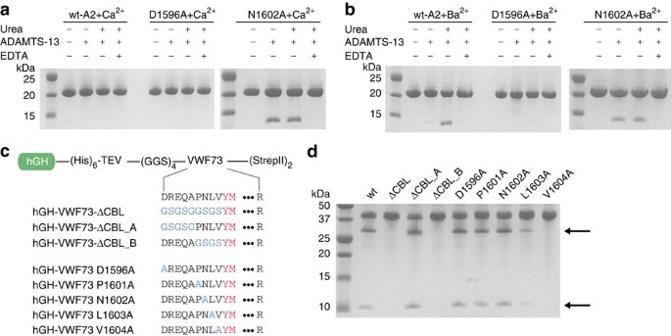Figure 4: VWF-A2 proteolysis by ADAMTS-13. (a) The recombinant wt-A2 or the calcium-binding-deficient mutants D1596A and N1602A were incubated with 6 nM ADAMTS-13 and 5 mM CaCl2, with and without 1.5 M urea. No cleavage is observed under these conditions for wt-A2 and D1596A, whereas the destabilized N1602A mutant is cleaved efficiently. (b) ADAMTS-13 cleaves wt-A2 and N1602A, but not D1596A if BaCl2replaces CaCl2. Because of divalent ion dependence of ADAMTS-13, no cleavage occurs in the presence of EDTA. (c) hGH–VWF73 fusion constructs. A (Gly–Gly–Ser)4linker was engineered between hGH and VWF73 to ensure that substrate cleavage is not influenced by vicinity of the hGH fusion. Substituted fragments of the α3β4-loop are highlighted in blue; the Tyr1605–Met1606 cleavage site is shown in magenta. (d) ADAMTS-13 cleavage of hGH–VWF73 constructs. VWF73 proteins with D1596A, P1601A and N1602A mutations are cleaved at similar rates as the wt sequence. Substrate specificity resides in the P3 and P2 residues Leu1603 and Val1604. Arrows indicate N- (upper arrow) and C-terminal (lower arrow) cleavage products. TEV: cleavage site for tobacco etch virus protease; CBL: calcium-binding loop. Figure 4: VWF-A2 proteolysis by ADAMTS-13. ( a ) The recombinant wt-A2 or the calcium-binding-deficient mutants D1596A and N1602A were incubated with 6 nM ADAMTS-13 and 5 mM CaCl 2 , with and without 1.5 M urea. No cleavage is observed under these conditions for wt-A2 and D1596A, whereas the destabilized N1602A mutant is cleaved efficiently. ( b ) ADAMTS-13 cleaves wt-A2 and N1602A, but not D1596A if BaCl 2 replaces CaCl 2 . Because of divalent ion dependence of ADAMTS-13, no cleavage occurs in the presence of EDTA. ( c ) hGH–VWF73 fusion constructs. A (Gly–Gly–Ser) 4 linker was engineered between hGH and VWF73 to ensure that substrate cleavage is not influenced by vicinity of the hGH fusion. Substituted fragments of the α 3 β 4 -loop are highlighted in blue; the Tyr1605–Met1606 cleavage site is shown in magenta. ( d ) ADAMTS-13 cleavage of hGH–VWF73 constructs. VWF73 proteins with D1596A, P1601A and N1602A mutations are cleaved at similar rates as the wt sequence. Substrate specificity resides in the P3 and P2 residues Leu1603 and Val1604. Arrows indicate N- (upper arrow) and C-terminal (lower arrow) cleavage products. TEV: cleavage site for tobacco etch virus protease; CBL: calcium-binding loop. Full size image Proteolysis of the unstructured hGH–VWF73 construct showed that the wt sequence and the D1596A and N1602A mutants are cleaved at similar rates ( Fig. 4d ). This indicates that the calcium-binding side chains of Asp1596 and Asn1602 do not directly contribute to substrate recognition. Our observation that the N1602A mutant is cleaved efficiently by ADAMTS-13 contrasts data by Zhou et al . [15] who, using a similar construct, observed no cleavage for this mutant. Although we cannot currently explain this discrepancy, it has been shown previously that deletion of α 3 β 4 residues Asp1596–Val1604 from an unstructured C-terminal A2 fragment prevents proteolysis of this fragment by ADAMTS-13 (refs 11 , 27 ), which suggests that this stretch of residues does contain elements that are essential for recognition by ADAMTS-13. To clarify this point, we systematically mutated the sequence that constitutes the α 3 β 4 -loop and β 4 -strand up to the scissile bond within the context of the hGH–VWF73 construct ( Fig. 4c ). Our data demonstrate that the residues critical for substrate recognition reside within the Pro1601–Val1604 sequence, as substitution of this sequence by GlySerGlySer abrogates cleavage completely, whereas substitution of residues Asp1596–Ala1600 by GlySerGlySerGly has no effect ( Fig. 4d ). Using individual alanine mutants of the Pro1601–Val1604 sequence, we find that the L1603A and V1604A mutations significantly affect the extent of cleavage, indicating that the P3 and, particularly, the P2 sites are important recognition elements for ADAMTS-13. On the basis of our data, we find no evidence for participation of Asn1602 at the P4 site, in recognition by ADAMTS-13. Instead our data suggest that its effect on the proteolysis rate is a consequence of reduced thermal stability because of loss of calcium binding. Calcium stabilizes an unfolding intermediate and promotes refolding The previous results show that calcium has an important role in protecting VWF from ADAMTS-13 cleavage under static, low shear stress conditions. These findings raise the question whether calcium might also have a role in high shear stress situations where the A2 domain can unfold. To address this issue, we used optical tweezers to apply tensile forces on single A2 molecules and followed their unfolding and refolding transitions in the presence or the absence of calcium. N-glycosylated A2 molecules containing an N-terminal (c-myc) 4 tag and a C-terminal biotin tag were immobilized on anti-myc-coated polystyrene beads and tethered to a second polystyrene bead via a ∼ 2500-bp DNA spacer by biotin–streptavidin interactions ( Fig. 5 ). We stretched and relaxed individual A2 molecules by displacing the bead on the pipette relative to the force-transducing bead in the optical trap and measured the resultant force versus extension curves at constant trap velocity. 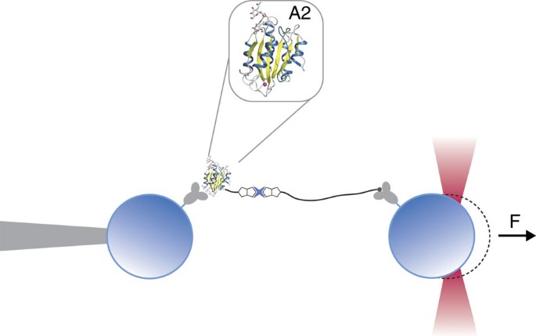Figure 5: Schematic illustration of the optical tweezers experiment. Single A2 domains (enlarged inset) are tethered between polystyrene beads that are held by a piezo-controlled micropipette and the optical trap. The tether includes a 2,500-bp DNA spacer to prevent unspecific bead–bead interactions. Figure 5: Schematic illustration of the optical tweezers experiment. Single A2 domains (enlarged inset) are tethered between polystyrene beads that are held by a piezo-controlled micropipette and the optical trap. The tether includes a 2,500-bp DNA spacer to prevent unspecific bead–bead interactions. Full size image First, we stretched individual tethers in the presence of EDTA to characterize the mechanical behaviour of A2 in the absence of calcium. At forces between 5 and 15 pN, we observed abrupt changes in extension, associated with a drop in force on the tether, which indicate unfolding transitions ( Fig. 6a,b ). To relate the observed extension changes to the sequence of the protein molecule, we used a serial worm-like chain (WLC) model [28] to fit our force-extension data. We obtained a total length increment (78±4 nm) that is in good agreement with the total length of A2 (196 residues) assuming a contour length contribution of 0.4 nm per residue [29] . The data suggest disruption of individual A2 molecules in a single unfolding transition, consistent with recent experiments performed with a similar construct [13] , [30] . 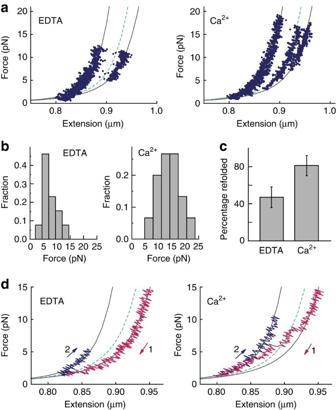Figure 6: Calcium modulates the folding and unfolding pathways of A2 under tensile force. (a) Representative force-extension data showing six unfolding experiments, without (left) and with (right) calcium. Grey lines represent WLC fits to the native and unfolded states. The green dashed line is the WLC fit to a subset of the data that populates an intermediate state. (b) Force distribution histograms for unfolding events with and without calcium obtained at a loading rate of 5 pN s−1. Mean unfolding forces are 7±3 pN (n=13) and 14±4 pN (n=15), respectively. (c) Probability to refold to the native state at zero load significantly increases in the presence of calcium (P<0.03). T-bars represent s.d. from counting statistics. (d) Relaxation traces (magenta) of A2 molecules without (left) or with (right) calcium show that A2 is able to refold against load only when calcium is present. The dashed line is the WLC fit to the intermediate observed during unfolding. Stretching traces observed after successful refolding are shown in blue. Figure 6: Calcium modulates the folding and unfolding pathways of A2 under tensile force. ( a ) Representative force-extension data showing six unfolding experiments, without (left) and with (right) calcium. Grey lines represent WLC fits to the native and unfolded states. The green dashed line is the WLC fit to a subset of the data that populates an intermediate state. ( b ) Force distribution histograms for unfolding events with and without calcium obtained at a loading rate of 5 pN s −1 . Mean unfolding forces are 7±3 pN ( n =13) and 14±4 pN ( n =15), respectively. ( c ) Probability to refold to the native state at zero load significantly increases in the presence of calcium ( P <0.03). T-bars represent s.d. from counting statistics. ( d ) Relaxation traces (magenta) of A2 molecules without (left) or with (right) calcium show that A2 is able to refold against load only when calcium is present. The dashed line is the WLC fit to the intermediate observed during unfolding. Stretching traces observed after successful refolding are shown in blue. Full size image Next, we repeated the experiments in the presence of calcium. Two marked differences were observed. The average force required for complete unfolding of A2 increased to 14±4 pN, a substantial (7±3 pN) and significant ( P <0.0001) increase of the resistance of the native state against tensile forces compared with the situation without calcium ( Fig. 6b ). In 59% of the observed transitions ( n =17), unfolding in the presence of calcium proceeded in a two-step manner via a well discernible intermediate that is stable against applied loads of up to 16 pN ( Fig. 6a ). The intermediate is consistent with a contour length that corresponds to 122±5 unfolded residues. In contrast, this intermediate is populated in only 21% of the unfolding events ( n =13) if calcium binding of A2 is suppressed by EDTA ( Supplementary Fig. S4a ); in all other events, unfolding under these conditions proceeded via a single transition. We investigated whether calcium also affects the folding pathway of A2. After each unfolding cycle, we relaxed the tether and waited for 5 s at zero force to allow the A2 domain to refold. Subsequently, the protein was stretched again to assess whether it had refolded, as identified by an unfolding force and length that are typical for the native state ( Supplementary Fig. S4b ). Again two pronounced differences were observed. With EDTA, native refolding was observed in 47% of the experiments ( n =17), whereas with calcium refolding occurred in 81% of the experiments ( n =16, P <0.03; Fig. 6c ). Assuming first-order kinetics, we roughly estimate that calcium increases the folding rate constant by six to seven-fold, which is a striking acceleration of the refolding process. Next, we found that 37% of the relaxation traces with calcium displayed clear deviations from the WLC model that indicate contraction of the polypeptide chain. Closer inspection suggests that at ∼ 5 pN, 71% of these traces transiently follow the same WLC curve that corresponds to the intermediate visited during unfolding, before displaying the native contour length at lower forces ( Fig. 6d ). Although the structural changes underlying the observed compaction under load remain unclear, our data suggest that folding of A2 proceeds via one or more intermediates that are induced by interactions with calcium. The increased probability to unfold via the intermediate in the presence of calcium suggests that calcium stabilizes the intermediate state. Intriguingly, the structure of the intermediate observed during unfolding does not seem to be a purely native substructure. The minimal substructure within the native state that contains all the native calcium interactions comprises 104 residues ( Fig. 1c ), which is significantly more than the 74±6 residues that we find experimentally when unfolding the intermediate. If refolding would occur through the same intermediate, this would suggest the formation of non-native contacts that are subsequently broken when folding to the native state. Overall, the single-molecule data indicate that calcium at physiological concentrations has a pronounced effect on the folding and unfolding pathway of A2 and support a dual functional role of calcium in both stabilizing A2 against mechanical unfolding and promoting refolding by acting as a folding cofactor that facilitates refolding against tensile load. In the circulation, where hydrodynamic forces are ubiquitous, a unique regulatory mechanism has evolved to achieve efficient adhesion to vascular lesions while avoiding excessive aggregation of platelets [31] . At the molecular level, this process involves the multimeric VWF molecule, which forms an avid binding platform for platelets. VWF responds to force on different levels. First, hydrodynamic shear forces induce a conformational change in VWF multimers [32] , [33] , thus revealing a hidden binding site and activating VWF for binding of platelets [34] . Second, the adhesive potential of VWF—which is determined by the size of its multimers—is negatively regulated by a feedback mechanism, in which critical shear forces lead to unfolding of the A2 domain, exposing a proteolytic cleavage site for ADAMTS-13. In this sense, the A2 domain of VWF is a mechanosensor that detects changes in hydrodynamic shear force to control platelet recruitment to lesions. Here we show that calcium binding to VWF-A2 critically affects its mechanosensing function by using a combination of structural, biochemical and single-molecule experiments. We find that the calcium-binding site visualized in our crystal structure stabilizes the native conformation of both the isolated A2 domain and A2 in its natural context. A2 binds calcium with micromolar affinity, implying that the metal-binding site in circulating VWF is saturated with calcium. Both the crystal structure and molecular dynamics simulations reveal that calcium binding restrains structural flexibility of the scissile-strand environment. Using a single-molecule approach, we find that calcium coordination markedly increases the resistance of A2 against mechanical unfolding, while at the same time accelerating native refolding and promoting folding in the presence of tensile forces by stabilizing an intermediate fold. These findings provide fundamental new insights in shear force sensing by VWF and its cleavage by ADAMTS-13. Calcium coordination, by stabilizing VWF-A2 in its native conformation, protects VWF-A2 from premature cleavage by ADAMTS-13 at low hydrodynamic forces, which is essential to preserve VWF multimers of sufficient size to elicit strong platelet interaction. The role of calcium in ADAMTS-13 proteolysis of VWF is janus-faced: it protects VWF, but at the same time activates ADAMTS-13 (refs 6 , 35 , 36 , 37 ). This concept explains previous observations on the effect of calcium and barium: barium can replace calcium as a cofactor of ADAMTS-13 activity [5] , but only marginally stabilizes A2 ( Fig. 3 ). The activating effect of barium on ADAMTS-13 far outweighs its stabilizing effect on A2 in static cleavage assays ( Fig. 4b ). Our data therefore resolve a persisting controversy concerning the dependence of ADAMTS-13 on calcium and barium for optimal activity in cleavage assays. Our single-molecule data indicate a central role of unfolding and refolding dynamics in VWF-A2 force sensing. A force sensor requires elastic elements that not only turn a signal 'on' once a certain threshold force is crossed but also turn it off again when the force drops below a critical value. Without calcium, A2 provides the first capability by unfolding beyond the unfolding force and exposing the cleavage site, but is poor at the second as it requires zero force for efficient refolding. Our study shows that calcium coordination fills this gap by promoting refolding despite an applied load, while at the same time increasing stability against forced unfolding. Such reversibility of switching enables a more dynamic and precise regulation by VWF-A2: once cleavage attenuates the shear force below a critical value, the remaining A2 domains can refold to maintain a balanced level of platelet recruitment. The data put a new perspective on the role of metal coordination in general. Although metal coordination is pervasive in proteins and its effect on equilibrium stability has been well studied, its potential role in shaping protein-folding pathways remains largely unexplored. Our results offer a first example of metal coordination that alters the folding and unfolding pathway of a protein under mechanical load. This pathway-level information may also help to explain the observed increases in refolding propensity, as our data suggest that refolding occurs via a calcium-induced intermediate state. Intermediate states can lower energy barriers and thus increase folding propensities, as has, for instance, been shown for filamin ddL4 in single-molecule studies [38] , [39] . It has recently been shown theoretically that length and force jumps observed with optical traps do not necessarily indicate the existence of a folding barrier in the absence of force, such as observed in bulk folding experiments [40] . Although folding at zero force is the pertinent physical condition for most proteins, A2, in contrast, is constantly subject to transient shear forces in its physiological environment and accordingly transitions across barriers of energy surfaces under load are of direct physiological relevance. Our data demonstrate that calcium modulates the collapse trajectory and enables A2 to refold against applied tensile forces. It would be of interest to know the precise structural changes underlying the transitions to and from the calcium-stabilized intermediate state observed during unfolding of A2, and to determine whether they can be cleaved by ADAMTS-13. The data provide intriguing hints. First, the observed calcium-induced unfolding intermediate is different from a VWF-A2 intermediate observed previously in the absence of calcium [13] , as well as from an intermediate suggested by molecular dynamics simulations in the presence of calcium [15] (and simulations performed by us; data not shown), which suggests that more than one intermediate structure might have a role. Second, although the observed refolding intermediate is calcium dependent, it does not contain the calcium coordination as found in the native structure, which indicates that non-native contacts are formed and broken during folding. Our data demonstrate, for the first time, that calcium coordination critically affects force sensing in VWF and suggests folding and unfolding equilibrium under tensile force to be a regulatory mechanism of VWF multimer size by ADAMTS-13 cleavage. Furthermore, it is intriguing to consider whether metal coordination also affects function and folding dynamics of other proteins. Protein expression and purification VWF residues 1,478–1,674 (A2), 1,261–1,674 (A1A2), 1,478–1,874 (A2A3) and 1,261–1,874 (A1A2A3) were expressed in HEK293-EBNA1-S cells. Culture supernatants were harvested 5 days after transfection and concentrated using a Quixstand hollow fiber system (GE Healthcare) before diafiltration into 25 mM HEPES (pH 7.8) and 0.5 M NaCl. A1 (residues 1,261–1,468) was expressed in Pichia pastoris as described previously [41] . Recombinant proteins were purified by Ni-NTA affinity chromatography, followed by proteolytic cleavage of the hexahistidine tag and further purified by ion exchange chromatography with MonoQ (GE Healthcare) in 20 mM HEPES, pH 7.8, with a 0–0.25 M NaCl gradient (A2, A1A2, A2A3 and A1A2A3) or MonoS (GE Healthcare) in 20 mM MES, pH 5.5, with a 0.2–0.3 M NaCl gradient (A1). N -glycans were trimmed by incubating proteins ( ∼ 1 mg ml −1 ) with EndoH f (NEB) in 0.1 M NaAc (pH 5.5) and 100 mM NaCl for 2 h at 37 °C. EndoH f was removed by affinity chromatography on amylose sepharose (NEB) in PBS. Proteins were finally purified by size exclusion chromatography in 15 mM HEPES (pH 7.5), 20 mM NaCl (100 mM for A1) and 1 mM CaCl 2 (A2, A2A3, A1A2 and A1A2A3). We noted that both mutant A2 constructs and wt-A2 in buffer without calcium are prone to aggregation during freeze–thawing or prolonged storage at 4 °C. The presence of aggregates affected thermal stability and ADAMTS-13 cleavage assays, and we therefore exclusively used material for which monodispersity was confirmed by analytical gel filtration immediately before the experiments. To study substrate specificity of ADAMTS-13, VWF73 constructs (residues 1,596–1,668) [27] with a C-terminal (StrepII) 2 tag were inserted into an expression vector encoding hGH containing a His tag and tobacco etch virus protease (TEV) cleavage site and including an additional (GlyGlySer)4 spacer between the TEV site and the VWF73 fragment. hGH–VWF73 fusion proteins were expressed in HEK293-EBNA1-S cells. Proteins were purified by Ni-NTA/StrepTactin tandem affinity chromatography, followed by size exclusion chromatography in 15 mM HEPES (pH 7.5) and 20 mM NaCl. Crystallization and refinement Crystals of A2 carrying a V1565L polymorphism ( Supplementary Fig. S5 ) were grown using hanging drop vapour diffusion at 292 K by mixing equal volumes of 9 mg ml −1 protein and reservoir solution. Within 24 h, crystals appeared as stacked needles in 0.1 M MMT (pH 4.3–4.7), 0.2 M (NH 4 ) 2 SO 4 , 18–20% (w/v) PEG2000 MME. Tiny needles (10×3×3 μm) were obtained by streak seeding with a cat whisker into 0.1 M MMT (pH 4.0–5.5), 0.15 M (NH 4 ) 2 SO 4 , 18–23% (w/v) PEG2000 MME. For cryoprotection, crystals were soaked in the crystallization condition supplemented with 20% (v/v) glycerol. Diffraction data were collected on the European Synchrotron Radiation Facility ID23-2 microfocus beamline and processed with XDS [42] and SCALA [43] . The crystal structure was solved using molecular replacement in PHASER [44] . Models were obtained from the human VWF-A3 domain (PDB accession code 1ATZ , ref. 20 ), with all side chains truncated to C β atoms and VWF-A2 (PDB accession code 3GXB , ref. 12 ). The structure was built in part using Arp/Warp [45] and completed manually in COOT [46] . The initial models were refined using PHENIX [47] and manual model building in COOT. Positional non-crystallographic symmetry constraints were imposed only during the initial steps of refinement. Calcium-ligand distances were initially restrained according to Harding [16] , [18] and refined unrestrained in the final steps of refinement. Table 1 summarizes data collection and refinement statistics. The crystal structure was validated with MolProbity [48] and showed 96.4 % of all residues in Ramachandran-favored and 99.3% in Ramachandran-allowed regions. There is one outlier, Ser1543, in all the three copies of the asymmetric unit, for which the density convincingly supports the modelled conformation. MD simulations All simulations and analysis were carried out using GROMACS version 3.3.3 (ref. 49 ). The OPLS-AA all-atom force field [50] and the TIP4P [51] water model were used. Proteins were solvated in cubic boxes with a minimum distance of 10 Å between solute and box edge. Sodium and chloride ions were added to an ionic strength of 150 mM and the appropriate number of additional ions was added to neutralize the system. The system was minimized by steepest descent minimization, and a subsequent 250-ps MD simulation with harmonic restraints on the protein main-chain atoms was carried out to equilibrate the solvent and ions. The final structure of this run served as starting structure for the subsequent MD simulations. Constant-pressure periodic boundary water box MD simulations were performed using particle-mesh Ewald summation [52] for long-range electrostatics. The systems were equilibrated for 5 ns before production runs. Temperature was kept constant at 300 K by coupling to the Nosé-Hoover thermostat, and a Parrinello–Rahman barostat was applied for pressure coupling. During the equilibration, the positional restraints on main-chain atoms were reduced stepwise. No restraints were applied in the production phase, and the equilibration part of the MD trajectories was not used for data analysis. During the final production runs, an integration step of 2.0 fs was used by applying the LINCS algorithm [53] to constrain bonds. The cutoff for van der Waals interactions was set to 10 Å during all simulations. Thermal denaturation assays Protein was dialysed into 50 mM HEPES (pH 7.5), 20 mM NaCl and 10 mM EDTA to remove divalent metal ions. Next, EDTA was removed by three successive dialysis steps into a 10,000-fold excess of 50 mM HEPES (pH 7.5) and 20 mM NaCl in Chelex100-filtered H 2 O (BioRad). All additives were dissolved in 50 mM HEPES (pH 7.5). A volume of 12.5 μl of a solution containing 500 ng protein was diluted in H 2 O with 5× Sypro Orange (Sigma-Aldrich) and immediately mixed with an equal volume of assay condition. All conditions were assessed in triplicate. Fluorescence increase was monitored on a MyiQ real-time PCR instrument (BioRad). Assays were performed over a temperature range of 15–90 °C using a ramp rate of 1 °C min −1 in steps of 0.5 °C. Fluorescence data from triplicate measurements were baseline corrected individually, and unfolding curves were normalized to maximum fluorescence to give fractional denaturation curves. The apparent T m was determined as the inflection point of a sigmoidal fit to the normalized fluorescence signal. The apparent K D was calculated from the concentration-dependent T m shift at varying calcium concentrations [26] . All calcium concentrations used for the K D calculations were corrected for a free calcium concentration of 1.0±0.1 (s.e.m.) μM as determined for the Chelex100-filtered buffer stock by titration with the chromophoric chelator 1,2-bis(2-amino-5-bromophenoxy)ethane- N,N,N′,N ′-tetraacetic acid (5,5′-dibromo-BAPTA) [54] . ADAMTS-13 cleavage assays Proteolysis assays were performed essentially as described by Pos et al . [55] . Briefly, 5 μl of 6 nM recombinant ADAMTS-13 was preincubated in 20 mM Tris (pH 7.8), 150 mM NaCl and 5 mM CaCl 2 (or BaCl 2 ) for 45 min at 37 °C before addition of 10 μM substrate (wt-, D1596A-, N1602A-A2 or hGH–VWF73). Similar reactions were also performed in the presence of 1.5 M urea. At these urea concentrations, ADAMTS-13 is active [1] , [2] , [56] . After 1 h, samples were analysed by SDS gel electrophoresis on 15% Tris-tricine gels. Optical tweezers A2 (residues 1,478–1,674) containing an N-terminal (c-myc) 4 tag and C-terminal Avi tag were expressed in HEK293-EBNA1 cells. Protein was purified by Ni-NTA affinity chromatography, followed by proteolytic cleavage of the His tag, biotinylated using BirA enzyme [57] and further purified by size exclusion chromatography in 20 mM HEPES (pH 7.5), 150 mM NaCl, containing 2.5 mM CaCl 2 (HBS-Ca) or 10 mM EDTA (HBS-EDTA). The double-stranded DNA linker, anti-dig and anti-c-myc beads were prepared as described [58] . Typically, 1 μl anti-dig beads were diluted in 10 μl HBS and mixed with 250 ng of digoxigenin- and biotin-labeled double-stranded DNA. Likewise, 1 μl of a suspension of anti-c-myc beads was mixed with 1–4 μl of 1 mg ml −1 A2. After 30 min incubation on a rotary mixer, beads were resuspended in 250 μl HBS-Ca or HBS-EDTA for use in the optical tweezers experiments. The optical tweezers setup was essentially as described elsewhere [58] . Detection of forces on the trapped microsphere was performed using back focal plane interferometry. Forces were recorded at 50 Hz. Trap stiffness was 169±24 pN μm −1 , and sensitivity was 2.74±0.24 V μm −1 . A piezo-nanopositioning stage (Physik Instrumente) was used to move the sample cell and micropipette at a speed of 50 nm s −1 , resulting in a pulling rate on the tethered A2 construct of ∼ 5 pN s −1 at unfolding. The microspheres were trapped in a flow chamber consisting of three parallel streams in laminar flow: one containing microspheres with A2, one containing microspheres with the DNA handle and a central buffer channel in which the measurements took place. Statistical significance of mean unfolding forces derived from force distributions was tested using Student's t -test. Barnard's exact test was applied for differences in refolding probability. Accession codes: Atomic coordinates and structure factors have been deposited with the Protein Data Bank under accession code 3ZQK . How to cite this article: Jakobi, A. J. et al . Calcium modulates force sensing by the von Willebrand factor A2 domain. Nat. Commun. 2:385 doi: 10.1038/ncomms1385 (2011).